Three-dimensional self-assembled photonic crystals with high temperature stability for thermal emission modification Selective thermal emission in a useful range of energies from a material operating at high temperatures is required for effective solar thermophotovoltaic energy conversion. Three-dimensional metallic photonic crystals can exhibit spectral emissivity that is modified compared with the emissivity of unstructured metals, resulting in an emission spectrum useful for solar thermophotovoltaics. However, retention of the three-dimensional mesostructure at high temperatures remains a significant challenge. Here we utilize self-assembled templates to fabricate high-quality tungsten photonic crystals that demonstrate unprecedented thermal stability up to at least 1,400 °C and modified thermal emission at solar thermophotovoltaic operating temperatures. We also obtain comparable thermal and optical results using a photonic crystal comprising a previously unstudied material, hafnium diboride, suggesting that refractory metallic ceramic materials are viable candidates for photonic crystal-based solar thermophotovoltaic devices and should be more extensively studied. The broad energy distribution of solar radiation is one of the fundamental factors limiting the efficiency of photovoltaic (PV) cells. Single-junction PV cells convert radiation to electricity most efficiently when that radiation has an energy comparable to the electronic band gap energy of the PV cell. Losses due to unabsorbed low-energy photons and thermalization of high-energy photons contribute to the limit in efficiency that can be achieved using a single-junction PV cell under solar irradiation (the Shockley Queisser limit) [1] . Multijunction cells provide increased efficiencies, but are challenging to manufacture at low cost. Another approach to high-efficiency solar energy harvesting is to convert the solar spectrum to near monochromatic radiation with energies comparable to the electronic band gap energy of a single-junction PV cell, minimizing losses due to unabsorbed photons and band edge thermalization, and enhancing the solar energy conversion efficiency. Solar thermophotovoltaic (sTPV) devices implement this approach by thermally coupling a broadband solar absorber with a spectrally selective thermal emitter, whose narrowed thermal emission can be more efficiently converted to electricity using a single-junction PV cell [2] , [3] , [4] , [5] , [6] , [7] , [8] . Strategies for broadband absorption of solar radiation are well understood [7] , [9] , [10] ; however, engineering spectral emissivity is challenging because emissivity is generally dominated by the fundamental optical properties of the constituent materials. The spectral conversion element must also be thermally stable and most calculations indicate the emitter temperature should be 1,000 °C or greater to be practical [3] , [4] , [5] , [6] , [7] , [11] , [12] . A small increase in the emitter-operating temperature ( T ) significantly increases the power output of the sTPV device (~ T 4 ) as predicted by the Stefan–Boltzmann law. Large emitter areas are also required because the emitted power scales with the emitter area, and fundamental thermodynamics require an emitter that has a substantially larger area as compared with the absorber [7] . Periodic structuring of materials on the order of the wavelength of light is one approach to spectrally alter emissivity [13] , [14] , [15] , [16] , [17] . Both two- [10] , [16] , [17] and three-dimensional (3D) architectures [13] , [14] , [15] can enhance or suppress thermal emission in desired frequency regimes yielding a spectral emissivity that can be more efficiently converted to electricity using a single-junction PV cell. 3D photonic crystals [18] , [19] , [20] are attractive because they may provide control of emissivity in all directions relative to the emitter, as well as more degrees of freedom for the design of structures with desired emission properties [12] , [13] , [14] , [21] . Two previous reports have demonstrated the potential of metallic 3D photonic crystals for thermal emission control [13] , [15] . Fleming et al . [13] reported modified thermal emission using a lithographically fabricated tungsten woodpile photonic crystal. The lithographic process is, however, complex, costly and slow, and the thermal stability of these architectures is unclear. Our group reported modified thermal emission using nickel photonic crystals; however, these structures degrade well below 1,000 °C (ref. 15 ). Self-assembled templates have been proposed as a means to achieve a scalable, large-area, high-quality, 3D photonic crystal emitter. Theoretical studies have indicated that the control of thermal emission using photonic crystals formed from self-assembled templates could rival or exceed that achieved using the 3D woodpile architecture [14] , [21] , [22] , [23] . Chemical vapour [24] , [25] , sol gel [23] , [26] or electrochemical [27] deposition methods have been used to deposit tungsten inside self-assembled templates in efforts to realize such structures. The thermal stability of the resulting materials, however, was limited in part by the quality and density of the deposited tungsten, and for this reason neither the emission nor any optical properties were discussed. Fabricating a thermally stable, large-area component that selectively emits thermal radiation in the near infrared remains a challenge for the realization of sTPV devices. Here we use self-assembled colloidal crystals to template the growth of a refractory material (tungsten deposited by atomic layer deposition (ALD) or hafnium diboride (HfB 2 ) deposited by chemical vapour deposition (CVD)) to generate photonic crystals that can serve as the selective thermal-emitting component of a sTPV device. This approach is quite general and other scalable templates (for example, those formed by interference lithography [28] ) could also be considered. Our tungsten structures are stable to at least 1,400 °C and suppress thermal emission of otherwise wasted low-energy photons at elevated temperatures. This combination of thermal stability and modified thermal emission has not been previously demonstrated for any 3D photonic crystal emitter. Comparable thermal and optical properties were obtained using HfB 2 photonic crystals, suggesting that refractory ceramic materials with metal-like optical properties, which are previously unexplored, are also useful for sTPV applications. Tungsten photonic crystal thermal stability Tungsten deposited by ALD, instead of CVD, is specifically advantageous for the conformal deposition of high-quality tungsten with a defined thickness [29] , [30] . Here tungsten photonic crystals were synthesized by conformal deposition on silica colloidal crystal templates using ALD. After ALD, tungsten was removed from the top of the structure by reactive ion etching, enabling removal of the silica template by chemical etching with hydrofluoric acid (HF), resulting in a tungsten-inverse colloidal crystal. The deposited tungsten was characterized using Auger electron spectroscopy (AES, Supplementary Fig. S1 ) and X-ray diffraction (XRD, Supplementary Fig. S2 ). The AES profile shows significant signal from silicon in the tungsten film (~5%), likely from the SiH 4 ALD precursor. The fluorine signal in the tungsten films (<0.6%) is likely from the WF 6 ALD precursor. These impurities are consistent with previous reports of tungsten ALD [31] , [32] , [33] . The ALD tungsten is amorphous as deposited. After annealing at 1,000 °C, the tungsten is crystalline and in the alpha phase. 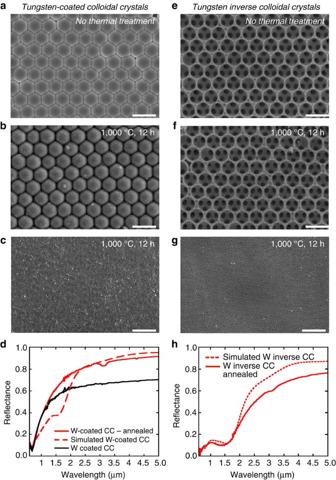Figure 1: SEM micrographs and reflectance properties of tungsten photonic crystals before and after annealing. The left column,a–dincludes data for tungsten (W)-coated colloidal crystals (CC). The right column,e–hincludes data for tungsten-inverse colloidal crystals. (a,e) Top-view micrographs, before annealing, of a tungsten-coated colloidal crystal and a tungsten-inverse colloidal crystal, respectively. Scale bars, 1 μm. (b,c) Top-view micrographs of a tungsten-coated colloidal crystal after annealing at 1,000 °C for 12 h. Scale bars, 1 and 10 μm, respectively. (f,g) Top-view micrographs of a tungsten-inverse colloidal crystal after annealing at 1,000 °C for 12 h. Scale bars, 1 and 10 μm, respectively. (d) Reflectance spectra of tungsten-coated colloidal crystals. The black spectrum is the measured reflectance of a tungsten-coated colloidal crystal before annealing. The red spectrum is the measured reflectance of the same sample after annealing at 1,000 °C for 12 h. The dashed red spectrum is the calculated reflectance of a tungsten-coated colloidal crystal. (h) Measured (solid red) and calculated (dashed red) reflectance spectra of a tungsten-inverse colloidal crystal. The measured sample was annealed at 1,000 °C for 12 h. Figure 1 includes the microstructure and optical properties of the tungsten photonic crystals after annealing to 1,000 °C for 12 h. The data in the left column correspond to tungsten-coated colloidal crystals and the right column contains data for the tungsten-inverse colloidal crystals. Both the tungsten-coated colloidal crystals and tungsten-inverse colloidal crystals retain their 3D periodic structure after they are annealed at 1,000 °C for 12 h and no significant cracking is observed. This result is unprecedented. All prior approaches resulted in micron-scale cracking and/or structural collapse at 1,000 °C (refs 23 , 24 , 25 , 26 , 27 ). We attribute this success to the tungsten ALD process, which may provide a denser tungsten material than previous methods, including those that utilized CVD, reducing material shrinkage and cracking at elevated temperatures. Figure 1: SEM micrographs and reflectance properties of tungsten photonic crystals before and after annealing. The left column, a – d includes data for tungsten (W)-coated colloidal crystals (CC). The right column, e – h includes data for tungsten-inverse colloidal crystals. ( a , e ) Top-view micrographs, before annealing, of a tungsten-coated colloidal crystal and a tungsten-inverse colloidal crystal, respectively. Scale bars, 1 μm. ( b , c ) Top-view micrographs of a tungsten-coated colloidal crystal after annealing at 1,000 °C for 12 h. Scale bars, 1 and 10 μm, respectively. ( f , g ) Top-view micrographs of a tungsten-inverse colloidal crystal after annealing at 1,000 °C for 12 h. Scale bars, 1 and 10 μm, respectively. ( d ) Reflectance spectra of tungsten-coated colloidal crystals. The black spectrum is the measured reflectance of a tungsten-coated colloidal crystal before annealing. The red spectrum is the measured reflectance of the same sample after annealing at 1,000 °C for 12 h. The dashed red spectrum is the calculated reflectance of a tungsten-coated colloidal crystal. ( h ) Measured (solid red) and calculated (dashed red) reflectance spectra of a tungsten-inverse colloidal crystal. The measured sample was annealed at 1,000 °C for 12 h. Full size image Heating the tungsten-coated colloidal crystals above 1,200 °C completely destroys the 3D structure ( Supplementary Fig. S3 ). Failure is most probably a result of tungsten sintering and concurrent template softening as silica has a glass transition temperature of ~1,200 °C. Similarly, tungsten-inverse colloidal crystals are also destroyed after heating to temperatures >1,200 °C, probably because of tungsten sintering ( Fig. 2a ). However, a protective coating of a refractory oxide (here 20 nm of hafnium dioxide, HfO 2 ) conformally deposited by ALD onto the tungsten-inverse colloidal crystals significantly enhances their high temperature stability [27] . As a result, we observe substantial retention of the 3D mesostructures even after annealing at 1,400 °C for 1 h ( Fig. 2b,c ). Although some of the fine structural features are slightly degraded, the overall 3D periodicity is retained and we observe no evidence of large-scale cracking ( Fig. 2c ). The structural integrity achieved on heating to 1,400 °C is unprecedented. We suspect optimization of the refractory coating may enable even greater thermal stability. 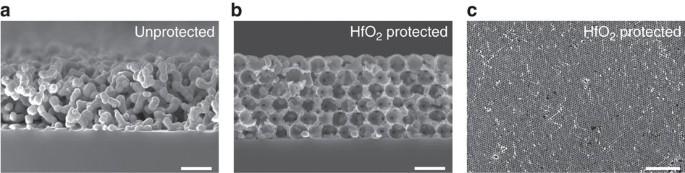Figure 2: SEM micrographs of tungsten-inverse colloidal crystals after annealing at temperatures above 1,000 °C. (a) Fracture cross-section micrograph of a tungsten-inverse colloidal crystal (unprotected) after heating to 1,200 °C for 1 h. Scale bar, 1 μm. (b) Fracture cross-section and (c) top-view micrographs of a tungsten-inverse colloidal crystal protected with HfO2after annealing at 1,400 °C for 1 h. Scale bars, 1 and 10 μm, respectively. Figure 2: SEM micrographs of tungsten-inverse colloidal crystals after annealing at temperatures above 1,000 °C. ( a ) Fracture cross-section micrograph of a tungsten-inverse colloidal crystal (unprotected) after heating to 1,200 °C for 1 h. Scale bar, 1 μm. ( b ) Fracture cross-section and ( c ) top-view micrographs of a tungsten-inverse colloidal crystal protected with HfO 2 after annealing at 1,400 °C for 1 h. Scale bars, 1 and 10 μm, respectively. Full size image Tungsten photonic crystal optical characterization The optical properties of the tungsten photonic crystals were probed by collecting reflectance ( R ) measurements using a Fourier transform infrared spectrometer (FTIR). Reflectance is commonly used to predict the spectral emissivity of a material because Kirchhoff’s law states that emission is equal to absorption, which is equal to 1- R . Materials that have a high reflectance at a given frequency will have a correspondingly low emissivity. Suppressed emissivity (high reflectance) in the infrared (IR) is important for a sTPV device because black body emission contains a large number of sub-electronic band gap photons that are not absorbed by a PV cell. As deposited, the tungsten-coated colloidal crystals exhibit low reflectance in the visible regime that sharply increases around 1 μm to 70% ( Fig. 1d , black spectrum). The high reflectance in the IR is observed until at least the limits of the detector (5 μm). After the samples are annealed at 1,000 °C for 12 h, the reflectance of the tungsten-coated colloidal crystals remains low in the visible and becomes enhanced in the IR, reaching a value of ~90% ( Fig. 1d , solid red spectrum). Crystallization on heating likely alters the optical properties of the tungsten material, and thus the photonic crystal. In general, the reflectance in the IR of the tungsten-inverse colloidal crystals is lower in intensity, and the transition from low reflectance to high reflectance is red shifted as compared with the tungsten-coated colloidal crystals. Figure 1h is the reflectance spectrum of a tungsten-inverse colloidal crystal after it was annealed at 1,000 °C for 12 h (solid red spectrum). After annealing the HfO 2 protected tungsten-inverse colloidal crystals at 1,400 °C for 1 h, the reflectance decreases in intensity ( Supplementary Fig. S4 ), probably because of the slight degradation of the structure ( Fig. 2 ). For reference, the reflectance spectrum of a flat tungsten film deposited by ALD is included in Supplementary Fig. S5 . The finite difference time domain (FDTD) method was used to calculate the expected reflectance spectra of these structures using optical constants of crystalline tungsten taken from the literature. For the tungsten-coated colloidal crystals annealed for 12 h at 1,000 °C, the general form of the simulated reflectance spectrum ( Fig. 1d , dashed red spectrum) approaches the measured reflectance spectrum ( Fig. 1d , solid red spectrum). The reflectance of the tungsten-inverse colloidal crystals as predicted by FDTD is included in Fig. 1h (dashed red spectrum) and the spectral shape closely matches the measured data (solid red spectrum). The measured reflectance is less than the calculated intensity, in particular at longer wavelengths; however, this result is not surprising, given the roughness of the top surface of the etched tungsten photonic crystal, which is not included in the simulation. Thermal emission measurements of the tungsten photonic crystals at elevated temperatures (900 °C) were conducted using a homebuilt emissometer to experimentally verify suppression of thermal emission at undesired energies. A detailed discussion of the thermal emission measurements can be found in the Methods section, and Supplementary Fig. S6 is a schematic of the emissometer. In brief, the samples were heated in vacuum to 900 °C and thermal emission was collected using a FTIR spectrometer. A calibrated black body standard was used as a reference to calculate the relative emissivity of the photonic crystals. 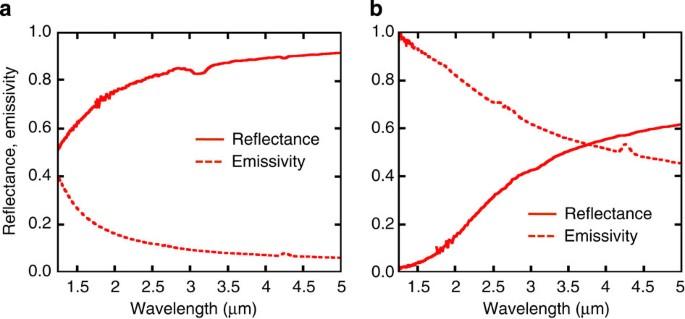Figure 3:Measured emissivity and reflectance of annealed tungsten photonic crystals. (a) Emissivity (dashed red) and reflectance (solid red) of a tungsten-coated colloidal crystal after annealing at 1,000 °C for 12 h. (b) Emissivity (dashed red) and reflectance (solid red) of a tungsten-inverse colloidal crystal, protected with HfO2, after annealing to 1,400 °C for 1 h. For both graphs, note that emissivity is approximately 1-R, as predicted by Kirchhoff’s law. Figure 3 shows the measured reflectance ( R ) and measured emissivity of a tungsten-coated colloidal crystal ( Fig. 3a ) that was previously annealed at 1,000 °C for 12 h and a tungsten-inverse colloidal crystal protected with HfO 2 ( Fig. 3b ) that was previously annealed at 1,400 °C for 1 h. As predicted from Kirchhoff’s law, the measured relative emissivity is very close to 1- R . The agreement between these two independent measurements of reflectance and emissivity provides an indication of the consistency of the data. Both structures exhibited suppressed thermal emission at long wavelengths. In any sTPV device, suppressed emission of long wavelength photons will result in fewer sub-electronic band gap photons arriving at the PV cell and thus less wasted energy. Figure 3: Measured emissivity and reflectance of annealed tungsten photonic crystals . ( a ) Emissivity (dashed red) and reflectance (solid red) of a tungsten-coated colloidal crystal after annealing at 1,000 °C for 12 h. ( b ) Emissivity (dashed red) and reflectance (solid red) of a tungsten-inverse colloidal crystal, protected with HfO 2 , after annealing to 1,400 °C for 1 h. For both graphs, note that emissivity is approximately 1-R, as predicted by Kirchhoff’s law. Full size image The power of thermal emission from a real material, at a given energy, cannot exceed the power emitted by a theoretical black body at the same temperature, T . Thus, maximum power output from a selective thermal emitter operating at temperature, T , is achieved when the spectral position of the allowed emission band coincides with the spectral position of the maximum in the black body spectrum for the same temperature, T . To achieve high-efficiency energy conversion, the PV material must efficiently convert light to electricity within that narrow band of allowed emission. 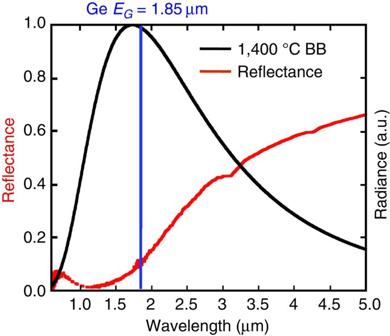Figure 4: Spectral alignment of TPV components. Reflectance of a tungsten-inverse colloidal crystal, protected with HfO2, annealed at 1,400 °C for 1 h (red spectrum) plotted with the theoretical black body emission at 1,400 °C (black spectrum). The blue line indicates the electronic band gap of germanium. Figure 4 shows that the peak emissivity (low reflection) of the HfO 2 -protected tungsten-inverse colloidal crystal is spectrally aligned with the maximum in theoretical black body emission at 1,400 °C and with the electronic band gap energy of germanium (1.85 μm, 0.67 eV), a low band gap energy PV material. As an emitter for TPV applications, our structures are spectrally tuned for operation at high temperature and spectrally aligned with common PV cells to achieve high-power and high-efficiency devices. Figure 4: Spectral alignment of TPV components. Reflectance of a tungsten-inverse colloidal crystal, protected with HfO 2 , annealed at 1,400 °C for 1 h (red spectrum) plotted with the theoretical black body emission at 1,400 °C (black spectrum). The blue line indicates the electronic band gap of germanium. Full size image HfB 2 photonic crystals To further maximize radiant power output, higher emitter temperatures than may be achievable with refractory metals would be desirable, and increases in the diversity of the optical properties beyond those provided by refractory metals would increase the available design space. Certain refractory ceramics, for example, some borides, nitrides and carbides, possess both metal-like optical properties and exceptional thermal stability [34] , [35] . Here using a similar process as demonstrated for the tungsten photonic crystals, for the first time, we fabricate a HfB 2 3D photonic crystal to investigate the possibility of refractory metallic ceramic compounds for sTPV applications. The HfB 2 photonic crystals were fabricated by conformal deposition on silica colloidal crystal templates using static CVD ( Supplementary Fig. S7 ). The deposited HfB 2 was characterized using AES ( Supplementary Fig. S8 ) and XRD ( Supplementary Fig. S9 ). The AES signal from oxygen within the film is ~0.5% and the carbon signal is ~1.5%. The deposited material is near stoichiometric and amorphous. After annealing at 1,000 °C for 12 h the material is crystalline. As deposited, the HfB 2 -coated colloidal crystals did not demonstrate high reflectance in the IR ( Fig. 5d , black spectrum). However, after annealing, the HfB 2 -coated colloidal crystals exhibit low reflectance in the visible and higher reflectance (60%) above around 1 μm ( Fig. 5d , red spectrum). Previous studies indicate that annealing low temperature deposited HfB 2 alters its optical properties [36] probably because of crystallization on heating ( Supplementary Fig. S9 ). The thermal stability of the HfB 2 photonic crystals is also presented in Fig. 5 . 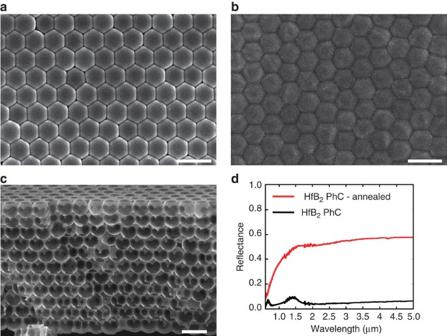Figure 5:SEM micrographs and reflectance properties of hafnium diboride photonic crystals before and after annealing. (a) Top-view micrograph of a HfB2-coated colloidal crystal before annealing. (b) Top-view micrograph of a HfB2-coated colloidal crystal after annealing at 1,000 °C for 12 h. (c) Fracture cross-section micrograph of a HfB2-inverse colloidal crystal after annealing at 1,000 °C for 12 h. (d) Reflectance spectra of a HfB2photonic crystal (PhC). The black spectrum is the measured reflectance of a HfB2-coated colloidal crystal before annealing. The red spectrum is the measured reflectance of a HfB2-coated colloidal crystal after annealing at 1,000 °C for 12 h. Scale bars, 1 μm. Figure 5a is a top-view scanning electron microscope (SEM) micrograph of a HfB 2 -coated colloidal crystal, as deposited. Figure 5b is a top-view SEM micrograph of a HfB 2 -coated colloidal crystal after it was annealed at 1,000 °C for 12 h. The 3D structure is preserved; however, there is evidence of larger-scale cracking after annealing ( Supplementary Fig. S10 ). Figure 5c is a fracture cross-section SEM micrograph of a HfB 2 -inverse colloidal crystal after annealing at 1,000 °C for 12 h. Above 1,000 °C, the HfB 2 samples were generally destroyed by oxidation, limiting our ability to do higher temperature studies, although significant care was taken to remove oxygen from the annealing environment. The intrinsic thermal stability of the HfB 2 photonic crystals is notably greater than previous reports of tungsten photonic crystals [23] , [24] , [25] , [26] , [27] , but does not yet match the stability of the HfO 2 -protected tungsten structures presented here. Better control of the oxygen partial pressure during annealing, possibly in conjunction with conformal protective coatings [27] or additives [37] could enhance the oxidative stability of these structures. Figure 5: SEM micrographs and reflectance properties of hafnium diboride photonic crystals before and after annealing . ( a ) Top-view micrograph of a HfB 2 -coated colloidal crystal before annealing. ( b ) Top-view micrograph of a HfB 2 -coated colloidal crystal after annealing at 1,000 °C for 12 h. ( c ) Fracture cross-section micrograph of a HfB 2 -inverse colloidal crystal after annealing at 1,000 °C for 12 h. ( d ) Reflectance spectra of a HfB 2 photonic crystal (PhC). The black spectrum is the measured reflectance of a HfB 2 -coated colloidal crystal before annealing. The red spectrum is the measured reflectance of a HfB 2 -coated colloidal crystal after annealing at 1,000 °C for 12 h. Scale bars, 1 μm. Full size image Materials challenges are limiting the development of useful 3D photonic crystal emitters for practical sTPV devices. Using a scalable process and two different material systems, we synthesized 3D photonic crystals that can shape the spectral emissivity and withstand extreme temperatures. Our tungsten photonic crystals are thermally stable up to 1,400 °C and stable up to 1,000 °C for at least 12 h. Large-area structures remain crack-free and we observed minimal change in the fine nanometre-scale organization of the 3D tungsten photonic crystals after being annealed. The thermal stability of these tungsten architectures is unprecedented and was achieved through high-quality material deposition and subsequent protection using a conformal refractory oxide coating. Although tungsten has been the most studied material to date for TPV applications, future research and development will likely expose limitations of tungsten, and conventional metals, in general. Initial investigations of HfB 2 photonic crystals with thermal stability up to at least 1,000 °C imply that the broader class of refractory metallic ceramic materials could be useful for TPV applications and should be further studied. These materials alone, or possibly in conjunction with conventional metallic materials, could enable superior thermal and optical performance of 3D photonic crystal emitters. The preservation of order and structural integrity at elevated temperatures enabled a direct measurement of thermal emission. Experimental measurements of thermal emissivity at 900 °C illustrate the desired suppression of thermal emission at long wavelengths. Corresponding reflectance data agree well with emissivity based on Kirchhoff’s law and can be adequately explained using FDTD simulations. Through careful control of the structure, our 3D photonic crystals preferentially emit thermal radiation in the near infrared regime, spectrally aligned to achieve maximum power and efficiency if implemented in a real TPV device. In summary, the combination of superior thermal stability and a direct measurement of modified thermal emission presented in this manuscript has not been previously demonstrated for a 3D photonic crystal emitter with feature sizes tuned for operation at high temperature and at frequencies required for TPV applications. Moreover, the materials and related structures presented in this manuscript may have an impact on other related areas, including thermal energy harvesting from waste heat, more efficient incandescent light sources, high-temperature catalysis and electrochemical energy storage. Colloidal crystal template fabrication Silica colloids were fabricated using the methods described by Stöber et al . [38] Colloidal crystals were assembled using previously published techniques [39] . Substrates (typically silicon or c-plane sapphire) were cleaned with piranha (3:1 H 2 SO 4 :H 2 O 2 by volume) before colloidal crystal growth. Caution: piranha is a strong oxidizing agent and should be handled with care. Tungsten photonic crystal fabrication Tungsten was conformally deposited on colloidal crystal templates using a homebuilt flow-tube ALD system at 215 °C and 0.6 Torr using nitrogen as a carrier gas flowing at 20 s.c.c.m. (50 nm, 125 cycles, 1 s pulse of WF 6 , 60 s hold, 60 s purge, 300 s pulse of SiH 4 and 120 s purge) [40] . Before tungsten ALD, 10 nm of aluminium oxide (Al 2 O 3 ) was deposited on the colloidal crystal template (90 cycles, 0.3 s pulse of trimethylaluminum, 20 s hold, 60 s purge, 0.3 s pulse of water, 20 s hold and 90 s purge). The Al 2 O 3 layer improves nucleation of tungsten during deposition. Template etching was achieved by first removing the top tungsten layer using a 20-s reactive ion etch (50 mTorr, 100 Watts, 4 s.c.c.m. O 2 , 16 s.c.c.m. SF 6 ). This overlayer removal exposed the silica template, which was subsequently etched using 5% HF diluted with ethanol. Caution: HF is extremely toxic and should be handled with appropriate personal protection and inside a fume hood. Hafnium oxide protective coatings were deposited by using a Savannah ALD from Cambridge Nanotech. HfB 2 photonic crystal fabrication A static CVD system, operating at high precursor pressures (15 Torr), was built to achieve conformal coatings on silica colloidal crystal templates. Hafnium borohydride (solid at room temperatures with a 15-Torr vapour pressure) was used as a single source precursor for HfB 2 CVD and was prepared in an inert atmosphere [36] , [41] , [42] . Equipment needed for the static CVD included a rough vacuum pump, ultra high purity argon, tube furnace, two glass tubes (0.75 inches in diameter connected by an on/off valve with ground glass joints). A schematic of the static CVD system is displayed in Supplementary Fig. S7 . One tube contained the solid precursor (precursor chamber), whereas the other contained the colloidal crystal template (sample chamber). Up to six templates were loaded into the sample chamber and coated simultaneously. Initially, the valve connecting the two chambers was closed, isolating the separate chambers. The precursor chamber was evacuated and left under vacuum. The sample chamber was evacuated and refilled with argon multiple times. In addition, the sample chamber was heated with a heat gun during cycling. After cycling, the valve between the chambers was opened, allowing gaseous hafnium borohydride to diffuse into the sample chamber and the pressure to reach the equilibrium vapour pressure of the precursor. The gaseous precursor was trapped in the sample chamber by closing the valve between the chambers. The sample chamber was heated in a tube furnace at 1 °C min −1 to 200 °C and held at temperature for 2 h. The resulting HfB 2 deposition was conformal and uniform in thickness throughout the bulk of the photonic crystal. After static CVD, template etching was achieved by first removing the top HfB 2 layer using a 2-h reactive ion etch (100 mTorr, 150 Watts, 4 s.c.c.m. O 2 , 16 s.c.c.m. CF 4 ). This overlayer removal exposed the silica template, which was subsequently etched using 5% HF diluted with ethanol and glycerol (60:40% by volume). Thermal annealing Thermal annealing experiments were conducted in a tube furnace from CM Industries, Inc. A 2-inch (outside diameter) mullite tube was used for all experiments. The tube was typically purged with ultra high purity argon for 2 h before annealing and continued to flow during annealing. Carbon felt from Merson USA was packed into the tube, upstream from the sample being annealed. This carbon acted as an oxygen getter to reduce the oxygen partial pressure at the sample. To further reduce the oxygen partial pressure at the sample during annealing, the samples were sandwiched between two sheets of tungsten foil from Sigma-Aldrich. The temperature was always ramped at a rate of 500 °C h −1 . Materials characterization Scanning electron micrographs were collected using a Hitachi S-4800 high-resolution field emission SEM. AES was conducted using a Physical Electronics PHI 660. Supplementary Fig. S1 is the AES depth profile of a tungsten film that was deposited on a silicon substrate using the same conditions described for photonic crystal fabrication. Al 2 O 3 was deposited by ALD (10 nm) on the silicon substrate before tungsten deposition. The aluminium and oxygen peaks observed around 670 s correspond to this Al 2 O 3 nucleation layer. The increasing silicon signal around 670 s, corresponds to the silicon substrate. Supplementary Fig. S8 is the AES depth profile of a HfB 2 film that was ~50 nm thick, deposited by static CVD. The rising silicon signal beginning around 280 s is probably because of the silicon substrate. XRD analysis was performed using a Philips X’pert MRD system with Cu Kα radiation and a nickel filter. The Al 2 O 3 peaks detected in the tungsten XRD pattern ( Supplementary Fig. S2 ) are present because of the sapphire substrate (c-plane). The silicon peaks in the HfB 2 XRD pattern are present because of the silicon substrate ( Supplementary Fig. S9 ). The broad peak at low angles present in both diffraction patterns correspond to the amorphous silica colloidal crystal template. Reflectance and thermal emission measurements Reflectance spectrums were collected using a Vertex 70 FTIR with a Bruker Hyperion microscope attachment. Data in the visible to 1.2 μm were collected using a × 10 glass microscope objective (numerical aperture (NA)=0.1), quartz beam splitter and a Si diode detector. Data from 1.2–1.8 μm were collected using a × 10 glass microscope objective (NA=0.1), quartz beam splitter and a liquid nitrogen-cooled InSb detector. Data for wavelengths greater than 1.8 μm were collected using a × 8.89 ZnSe objective (NA=0.08), CaF 2 beam splitter and a liquid nitrogen-cooled InSb detector. The experimental system used to measure thermal emission (emissometer) is schematically described in Supplementary Fig. S6 . This emissometer consisted of a hot stage (HeatWave Labs, Model 104863) in a vacuum chamber, focusing optics, a black body reference source and a FTIR spectrometer (Thermo Scientific Nicolet 6700). The black body reference source and temperature controller were purchased from Boston Electronics (IR-564 and IR-301, respectively). Samples were mounted on the heating stage inside the vacuum chamber. The vacuum system base pressure of 1 × 10 −6 Torr was achieved using a turbo molecular pump. This vacuum level was sufficient to prevent sample oxidation during heating for short times. Light emitted from the sample excited the vacuum chamber through a CaF 2 window, reflected off of two gold parabolic mirrors (PM1 and PM3), passed through an interferometer with a CaF 2 beam splitter and was finally collected by a mercury cadmium telluride detector ( Supplementary Fig. S6a ). An aperture (APT) was placed in the optical path, between the two gold mirrors. This aperture was used to control the spot size measured from the sample. A laser was used to align the mirrors on the appropriate collection area. The black body reference source was mounted opposite to and facing the vacuum chamber. PM1 was mounted on a translatable stage with a second, identical gold parabolic mirror (PM2). PM1 and PM2 were mounted at 90° with respect to each other. Translating the stage towards the black body reference source aligned PM1 with PM3 for collection of thermal emission from a heated sample in the vacuum chamber ( Supplementary Fig. S6a ). Translating the stage towards the vacuum chamber aligned PM2 with PM3 for collection of thermal emission from the black body reference source ( Supplementary Fig. S6b ). In the two different configurations, the distance from PM1 to the surface of the heat stage was identical to the distance from PM2 to the black body source. To calculate the relative emissivity, first, the spectral radiance of the black body reference source was collected at one temperature, S BB,Measured ( λ,T ). A transfer function (equation (1)) of the emissometer was calculated by dividing the theoretical black body spectrum, L BB,Theory ( λ,T ), by the measured spectrum, S BB,Measured ( λ,T ). The transfer function was independent of temperature and was used to accurately calculate the true spectral radiance of our photonic crystals, L PhC (λ,T) (equation (2)). The relative emissivity of our photonic crystals was the ratio of L PhC (λ,T) to L BB,Theory (λ,T) (equation (3)). Appropriate normalization using the methods described above requires an accurate measurement of sample temperature. Here we deposited carbon black on the edge of the substrate of the photonic crystals that were studied. Carbon has a relative emissivity of 0.85 that does not vary significantly within the spectral region of interest. Therefore, the emission spectrum of the carbon black has the same spectral shape as that of the black body. The raw emission from the carbon black was collected just before collecting the raw emission data from the photonic crystal on the same substrate. The actual temperature of the carbon black was calculated from the shape of the emission spectrum of the carbon black. A more detailed discussion of the calibration procedure can be found in a separate publication [43] . It was assumed that the temperature of the photonic crystal on the same substrate was at the same temperature as the carbon black. FDTD simulations The fabricated photonic crystals were computationally studied using the FDTD method. Please refer to other sources for a detailed description of FDTD and the other computational methods for photonic crystals [19] , [44] , [45] . FDTD simulations were done using free software, MIT Electromagnetic Equation Propagation. Simulations were only done for tungsten photonic crystals because the dielectric constant data for HfB 2 are not well known. The tungsten photonic crystals were represented using appropriate dielectric constant data for tungsten [46] . Both real and imaginary parts of the dielectric constant were used because tungsten is absorptive. Simulations for tungsten photonic crystals accounted for the Al 2 O 3 nucleation layer that was deposited before tungsten deposition. The simulations accounted for the top layer of tungsten on the tungsten-coated colloidal crystals. Simulations did not include this top tungsten overlayer for the tungsten-inverse colloidal crystals because this overlayer was removed by reactive ion etching. How to cite this article: Arpin, K. A. et al . Three-dimensional self-assembled photonic crystals with high temperature stability for thermal emission modification. Nat. Commun. 4:2630 doi: 10.1038/ncomms3630 (2013).